Human CLPP reverts the longevity phenotype of a fungalClpPdeletion strain Mitochondrial maintenance crucially depends on the quality control of proteins by various chaperones, proteases and repair enzymes. While most of the involved components have been studied in some detail, little is known on the biological role of the CLPXP protease complex located in the mitochondrial matrix. Here we show that deletion of PaClpP , encoding the CLP protease proteolytic subunit CLPP, leads to an unexpected healthy phenotype and increased lifespan of the fungal ageing model organism Podospora anserina . This phenotype can be reverted by expression of human ClpP in the fungal deletion background, demonstrating functional conservation of human and fungal CLPP. Our results show that the biological role of eukaryotic CLP proteases can be studied in an experimentally accessible model organism. Mitochondria are organelles of eukaryotic organisms that are involved in a number of vital processes, including the assembly of iron/sulphur clusters, biosynthesis of lipids and amino acids and the generation of ATP via oxidative phosphorylation. Therefore, it is not surprising that mitochondrial dysfunction is associated with numerous adverse phenomena such as ageing [1] , [2] , [3] or degenerative diseases like Parkinson’s and Alzheimer’s disease [4] . To maintain a functional population of mitochondria, a complex network of quality control pathways is active [1] , [2] , [3] . In this network, protein quality control is fundamental. In the mitochondrial matrix of most eukaryotic organisms, two soluble AAA+ (ATPase associated with diverse cellular activities) serine proteases termed LON and CLPXP are located. While the former is a homo-oligomeric complex with each subunit containing a protease and chaperone domain [5] , CLPXP is a hetero-oligomeric complex consisting of individual CLPP proteolytic and CLPX chaperone subunits [6] . The cellular function of LON proteases, including their relevance for ageing processes, has been studied in some detail in a number of eukaryotic models [7] , [8] , [9] , [10] , [11] , [12] . In contrast, in part because of the lack of suitable model organisms, data on the biological role of the mitochondrial CLPXP protease complex, aside from its implied function in the so-called ‘mitochondrial unfolded protein response’ [13] , [14] , [15] , is scarce and to date no physiological substrates of any eukaryotic CLP protease have been identified. The filamentous ascomycete P. anserina which, in contrast to other filamentous fungi, is characterized by a limited lifespan, displays a clear mitochondrial aetiology of ageing and has been extensively investigated to unravel the molecular basis of ageing processes [16] . Recent work demonstrated a clear impact of mitochondrial protein quality control on the regulation of lifespan and stress adaptation in this model organism [10] , [12] , [17] . In the present study, we investigated the effects of deleting the gene encoding the CLP protease proteolytic subunit CLPP in P. anserina . Unexpectedly, the PaClpP deletion strain is viable and characterized by an extended lifespan without any distinct impairment. We further demonstrate that the longevity phenotype can be reverted by expression of human ClpP , thus identifying P. anserina as a promising in vivo model to study the biological role of the poorly characterized mitochondrial CLPXP protease complex. In silico identification of CLP protease components While CLPP is absent in several lower eukaryotes, including the yeasts Saccharomyces cerevisiae and Schizosaccharomyces pombe [6] , the genome of P. anserina codes for a CLPP homologue, as well as for homologues of the CLP chaperones CLPA, CLPB and CLPX ( http://podospora.igmors.u-psud.fr ). With the exception of the chaperone PaCLPA, all proteins have a predicted probability for mitochondrial localization of >90%. PaCLPP displays the expected distribution of the canonical catalytic residues (Ser, His and Asp) and is highly conserved compared to CLPP from other species, sharing about 60% similarity with the homologues from human, Caenorhabditis elegans and Escherichia coli ( Fig. 1a ). The deduced PaCLPP pre-protein is composed of 254 amino acids and contains a putative mitochondrial targeting sequence. After import into mitochondria, cleavage of the mitochondrial targeting sequence is expected to lead to a mature protein of ~25 kDa. 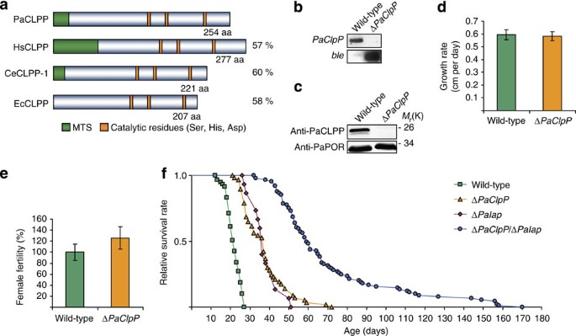Figure 1:Deletion ofClpPinP. anserinaextends the healthy lifespan at 27 °C. (a) The CLPP homologues fromP. anserina,Homo sapiens,C. elegansandE. colidisplay a conserved distribution of the canonical catalytic residues Ser, His and Asp. Additionally, all eukaryotic CLPPs contain a mitochondrial targeting sequence (MTS). The length of the different CLPP homologues varies from 207 amino acids inE. colito 277 amino acids inH. sapiens. The amino-acid sequence of PaCLPP shares 57%, 60% and 58% similarity with that of HsCLPP, CeCLPP-1, and EcCLPP, respectively. (b) Southern blot analysis ofHindIII digested genomic DNA from wild-type and ΔPaClpP. ThePaClpP-specific hybridization probe detects the 4995-bp fragment containingPaClpPonly in wild-type genomic DNA. A 2454-bp fragment containing the phleomycin resistance gene (ble) is detected by able-specific hybridization probe only in genomic DNA of ΔPaClpP. (c) Western blot analysis of mitochondrial protein extracts from wild-type and ΔPaClpP. The PaCLPP-specific antibody detects the ~25-kDa PaCLPP monomer only in the wild-type sample. PaPORIN (PaPOR) was detected as a loading control. (d) Growth rate of wild-type (0.60±0.04;n=59) and ΔPaClpP(0.58±0.04;n=55;P=0.07 by two-tailed Wilcoxon rank-sum test) isolates at 27 °C. Data given in parentheses are mean growth rate±s.e. in centimetres per day. (e) Female fertility of wild-type (100±14.7;n=11) and ΔPaClpP(126.1±20.3;n=11;P=0.26 by two-tailed Wilcoxon rank-sum test) isolates at 27 °C. Data given in parentheses are mean female fertility±s.e. in percentage. (f) Lifespan of wild-type (21.7±0.5;n=59), ΔPaClpP(37.1±1.5;n=57;P=5.8E-18), ΔPaIap(37.9±1.8;n=15;P=2.7E-09) and ΔPaClpP/ΔPaIap(70.6±3.4;n=90;P=8.5E-25) isolates at 27 °C. Data given in parentheses are mean lifespan±s.e. in days.P-values were determined in comparison with the wild-type sample by two-tailed Wilcoxon rank-sum test. Figure 1: Deletion of ClpP in P. anserina extends the healthy lifespan at 27 °C. ( a ) The CLPP homologues from P. anserina , Homo sapiens , C. elegans and E. coli display a conserved distribution of the canonical catalytic residues Ser, His and Asp. Additionally, all eukaryotic CLPPs contain a mitochondrial targeting sequence (MTS). The length of the different CLPP homologues varies from 207 amino acids in E. coli to 277 amino acids in H. sapiens . The amino-acid sequence of PaCLPP shares 57%, 60% and 58% similarity with that of HsCLPP, CeCLPP-1, and EcCLPP, respectively. ( b ) Southern blot analysis of Hin dIII digested genomic DNA from wild-type and Δ PaClpP . The PaClpP -specific hybridization probe detects the 4995-bp fragment containing PaClpP only in wild-type genomic DNA. A 2454-bp fragment containing the phleomycin resistance gene ( ble ) is detected by a ble -specific hybridization probe only in genomic DNA of Δ PaClpP . ( c ) Western blot analysis of mitochondrial protein extracts from wild-type and Δ PaClpP . The PaCLPP-specific antibody detects the ~25-kDa PaCLPP monomer only in the wild-type sample. PaPORIN (PaPOR) was detected as a loading control. ( d ) Growth rate of wild-type (0.60±0.04; n =59) and Δ PaClpP (0.58±0.04; n =55; P =0.07 by two-tailed Wilcoxon rank-sum test) isolates at 27 °C. Data given in parentheses are mean growth rate±s.e. in centimetres per day. ( e ) Female fertility of wild-type (100±14.7; n =11) and Δ PaClpP (126.1±20.3; n =11; P =0.26 by two-tailed Wilcoxon rank-sum test) isolates at 27 °C. Data given in parentheses are mean female fertility±s.e. in percentage. ( f ) Lifespan of wild-type (21.7±0.5; n =59), Δ PaClpP (37.1±1.5; n =57; P =5.8E-18), Δ PaIap (37.9±1.8; n =15; P =2.7E-09) and Δ PaClpP /Δ PaIap (70.6±3.4; n =90; P =8.5E-25) isolates at 27 °C. Data given in parentheses are mean lifespan±s.e. in days. P -values were determined in comparison with the wild-type sample by two-tailed Wilcoxon rank-sum test. Full size image Deletion of PaClpP extends lifespan To investigate the biological role of the mitochondrial CLPXP protease complex in P. anserina , we analysed a PaClpP deletion strain (Δ PaClpP ), which was generated in the course of an earlier study demonstrating that overexpression of the gene encoding the mitochondrial LON protease homologue PaLON1 in P. anserina results in robust lifespan extension [10] . In this context, the Δ PaClpP strain served as a control to assess the contribution of PaCLPP to the mitochondrial matrix serine protease activity but was not further characterized. Here we report this characterisation. After verification of Δ PaClpP by Southern blot analysis ( Fig. 1b ), absence of the protein in the deletion strain was confirmed by western blot analysis ( Fig. 1c ). Under standard growth conditions at 27 °C and constant light, the PaClpP deletion strain displayed no impairments of its vital functions, that is, growth rate and female fertility ( Fig. 1d ) and was morphologically indistinguishable from the wild-type. Furthermore, susceptibility of Δ PaClpP to various oxidative stressors thought to impair mitochondrial and/or cellular protein homoeostasis, including paraquat, copper sulphate and H 2 O 2 , as well as against dithiothreitol-induced endoplasmic reticulum (ER) stress was unchanged ( Supplementary Fig. S1 ). Remarkably, compared with the wild-type ( n =59), lifespan of Δ PaClpP ( n =57) was found to be significantly increased (mean lifespan:+71%, maximum lifespan:+167%; P =5.8E-18 by two-tailed Wilcoxon rank-sum test; Fig. 1f ). This result, though counter-intuitive at first glance, is reminiscent of the healthy longevity phenotype resulting from the deletion of PaIap , encoding the membrane-bound mitochondrial i -AAA protease in P. anserina [17] . Δ PaClpP longevity is independent of i -AAA and LON protease The observation that both Δ PaClpP and the PaIap deletion strain (Δ PaIap ) are long-lived at 27 °C prompted us to investigate whether these proteases might be involved in the same molecular pathways regulating lifespan. To this end, we generated a double mutant (Δ PaClpP /Δ PaIap ) in which both genes, that is, PaClpP and PaIap , are deleted ( Supplementary Fig. S2 ) and analysed its lifespan in comparison with the wild-type and the respective single deletion strains ( Fig. 1f ). A lifespan extension similar to that of Δ PaClpP was verified for Δ PaIap (mean lifespan:+74%, maximum lifespan:+89%; n =15), corresponding to the results obtained in an earlier study [17] . Interestingly, lifespan of the double deletion strain ( n =89) was even further increased (mean lifespan:+225%, maximum lifespan+530%) and significantly longer than that of either Δ PaClpP ( P =3.1E-17 by two-tailed Wilcoxon rank-sum test) or Δ PaIap ( P =4.2E-08 by two-tailed Wilcoxon rank-sum test). This additive lifespan extending effect following the concomitant deletion of PaClpP and PaIap suggests at least two possible scenarios: absence of the encoded components influences pathways acting in parallel to promote longevity or lack of either PaIAP or PaCLPP causes mild mitochondrial stress, an effect which is exacerbated in the double deletion strain, thereby activating common downstream pathways that are responsible for the observed extension of lifespan. In addition, to examine the epistatic relationship between PaClpP and PaIap in more detail, we analysed the lifespans and growth rates of the single and double deletion strains at 37 °C ( Supplementary Fig. S3 ). While deletion of PaIap had already been demonstrated to result in a pronounced heat-sensitive phenotype [17] , the PaClpP deletion strain displayed only a minor impairment of fitness at elevated temperatures. Interestingly, heat stress sensitivity of the Δ PaClpP /Δ PaIap double deletion strain was slightly increased compared with either single deletion strain. This observation argues for potentially overlapping functions of PaCLPP and PaIAP in a cellular heat stress response in P. anserina . As it was previously reported that overexpression of the gene coding for the P. anserina LON protease homologue PaLON1 led to an increase in healthspan similar to that of Δ PaClpP [10] , we also investigated whether the deletion strain’s longevity phenotype can be accounted for by a compensatory upregulation of this protease. Both CLPXP and LON are soluble proteases located in the mitochondrial matrix and it is thus well conceivable that they possess overlapping substrate specificities and may at least partially be able to compensate for dysfunction or even loss of each other. Yet, we observed no significant change in the relative PaLON1 protein abundance in mitochondrial protein extracts from the PaClpP deletion strain ( n =6) when compared with those of the wild-type strain ( n =6; P =0.63 by two-tailed Student’s t -test; Supplementary Fig. S4 ), suggesting that PaLON1 does not have a major role in the extended lifespan of Δ PaClpP . Human CLPP reverts the Δ PaClpP longevity phenotype Having demonstrated that deletion of PaClpP is non-lethal and leads to a specific phenotype, we asked the question of whether or not this phenotype can be reverted by heterologous expression of a construct coding for human CLPP. To ensure stable expression of the transgene, a vector containing the full-length open reading frame (ORF) of the human ClpP complementary DNA (cDNA) under control of a constitutive, P. anserina -specific promoter was constructed and subsequently transformed into protoplasts of the PaClpP deletion strain. The resulting transformants were verified by Southern blot analysis and two independent transformants (Δ PaClpP / HsClpP _OEx1 and 2), each with a single integration of the vector into their genome, were selected for subsequent experiments ( Supplementary Fig. S5 ). Western blot analysis of mitochondrial protein extracts from Δ PaClpP / HsClpP _OEx1 with an HsCLPP-specific antibody confirmed the presence of mature HsCLPP with an apparent molecular mass of ~26 kDa in mitochondria of the transgenic mutant strain ( Fig. 2a ). 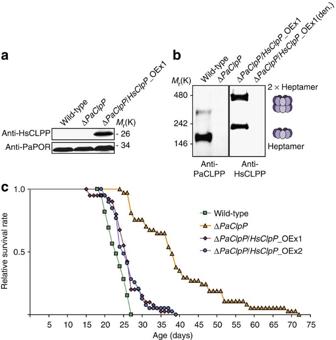Figure 2:Heterologous expression of humanClpPcomplements the longevity phenotype of ΔPaClpP. (a) Representative western blot analysis of mitochondrial protein extracts from wild-type, ΔPaClpPand ΔPaClpP/HsClpP_OEx1. The HsCLPP-specific antibody detects the ~26 kDa HsCLPP monomer only in the ΔPaClpP/HsClpP_OEx1 sample. PaPORIN (PaPOR) was detected as a loading control. (b) Western blot analysis of the same mitochondrial protein extracts as in (a) following BN-PAGE. Incubation of the western blot membrane with a PaCLPP-specific antibody visualized two oligomers with apparent molecular masses of ~170 and 340 kDa in the wild-type sample. In the ΔPaClpP/HsClpP_OEx1 sample, two distinct oligomers with apparent molecular masses of ~220 and 440 kDa were detected after incubation with an HsCLPP-specific antibody. Additionally, the ΔPaClpP/HsClpP_OEx1 (den.) sample was heat denatured for 10 min at 95 °C, after which the HsCLPP oligomers could not be detected anymore. (c) Lifespan of wild-type (23.3±0.4;n=39), ΔPaClpP(39.8±1.9;n=37;P=7.2E-13), ΔPaClpP/HsClpP_OEx1 (26.2±0.7;n=40;P=6.8E-04) and ΔPaClpP/HsClpP_OEx2 (26.2±0.7;n=39;P=2.5E-03) isolates at 27 °C. Data given in parentheses are mean lifespan±s.e. in days.P-values were determined in comparison with the wild-type sample by two-tailed Wilcoxon rank-sum test. Figure 2: Heterologous expression of human ClpP complements the longevity phenotype of Δ PaClpP. ( a ) Representative western blot analysis of mitochondrial protein extracts from wild-type, Δ PaClpP and Δ PaClpP / HsClpP _OEx1. The HsCLPP-specific antibody detects the ~26 kDa HsCLPP monomer only in the Δ PaClpP / HsClpP _OEx1 sample. PaPORIN (PaPOR) was detected as a loading control. ( b ) Western blot analysis of the same mitochondrial protein extracts as in ( a ) following BN-PAGE. Incubation of the western blot membrane with a PaCLPP-specific antibody visualized two oligomers with apparent molecular masses of ~170 and 340 kDa in the wild-type sample. In the Δ PaClpP / HsClpP _OEx1 sample, two distinct oligomers with apparent molecular masses of ~220 and 440 kDa were detected after incubation with an HsCLPP-specific antibody. Additionally, the Δ PaClpP / HsClpP _OEx1 (den.) sample was heat denatured for 10 min at 95 °C, after which the HsCLPP oligomers could not be detected anymore. ( c ) Lifespan of wild-type (23.3±0.4; n =39), Δ PaClpP (39.8±1.9; n =37; P =7.2E-13), Δ PaClpP / HsClpP _OEx1 (26.2±0.7; n =40; P =6.8E-04) and Δ PaClpP / HsClpP _OEx2 (26.2±0.7; n =39; P =2.5E-03) isolates at 27 °C. Data given in parentheses are mean lifespan±s.e. in days. P -values were determined in comparison with the wild-type sample by two-tailed Wilcoxon rank-sum test. Full size image Next, we examined whether HsCLPP forms functional oligomers in the mitochondria of P. anserina . The proteolytic core of the mitochondrial CLPXP protease complex is composed of two heptameric CLPP rings, which congregate to form a self-compartmentalised, cylindrical structure reminiscent of the 20S proteasome core particle. Only if HsCLPP were able to form this structure inside the fungal mitochondria, complementation of the deletion strain could be expected. To detect possible oligomers, mitochondrial protein extracts from Δ PaClpP / HsClpP _OEx1 were solubilised with the mild detergent digitonin and separated by blue native-polyacrylamide gel electrophoresis (BN-PAGE) [18] . After western blotting and incubation with an HsCLPP-specific antibody, two distinct oligomers could be detected in the Δ PaClpP / HsClpP _OEx1 sample ( Fig. 2b ). The apparent molecular mass ratio of these two oligomers was 1:2, as expected for the single heptameric CLPP ring and the CLPP proteolytic core cylinder formed by two such heptamers. After heat denaturation of the Δ PaClpP / HsClpP _OEx1 sample the signals disappeared, confirming the presence of bona fide HsCLPP oligomers inside mitochondria of the fungal transformants. However, the oligomers appeared roughly 20% larger than one would expect from calculating their molecular mass based on that of a single HsCLPP monomer. This apparent discrepancy can most likely be attributed to the migration of proteins during BN-PAGE being significantly influenced by their native shape, their intrinsic charge and the amount of bound Coomassie dye [19] . As an additional control, the western blot membrane was incubated with a PaCLPP-specific antibody, thereby visualizing endogenous PaCLPP oligomers in the mitochondrial protein extract from the wild-type strain. The apparent molecular mass of these oligomers was more in accord with their theoretically calculated size. Finally, lifespans of the transgenic Δ PaClpP / HsClpP _OEx mutant strains were analysed in comparison with their parental strain Δ PaClpP and the wild-type ( Fig. 2c ). The PaClpP deletion strain ( n =37) consistently showed an increase in its lifespan (mean lifespan:+71%, maximum lifespan:+167%) compared with the wild-type ( n =39; P =7.2E-13 by two-tailed Wilcoxon rank-sum test). Strikingly, lifespan of the two independent strains Δ PaClpP / HsClpP _OEx1 ( n =40) and 2 ( n =39) was only slightly longer than that of the wild-type (mean lifespan:+12%, maximum lifespan:+44%) and significantly reduced compared with Δ PaClpP (Δ PaClpP / HsClpP _OEx1: P =9.5E-10, Δ PaClpP / HsClpP _OEx2: P =2.4E-09 by two-tailed Wilcoxon rank-sum test). This almost complete reversion of Δ PaClpP ’s pronounced longevity phenotype by HsCLPP clearly argues for the capability of human CLPP to provide the in vivo functions of PaCLPP and thus demonstrates the functional conservation of CLPP from fungi to humans. The biological role of eukaryotic CLP proteases is as yet only poorly understood. Unfortunately, the unicellular ascomycete S. cerevisiae , the most thoroughly studied and accessible eukaryotic model organism [20] , lacks a CLPP homologue [6] and thus is not suitable to investigate eukaryotic CLP proteases. Strikingly, the genome of the filamentous ascomycete P. anserina encodes a CLPP homologue, as well as a homologue of the mitochondrial CLP chaperone CLPX. Our results demonstrate that deletion of PaClpP and thus ablation of mitochondrial CLPXP protease activity leads to a dual phenotype, that is, an extension of the healthy lifespan under standard growth conditions but slightly impaired fitness at elevated temperatures. Very similar effects have previously been observed in a PaIap deletion strain [17] . As the concomitant deletion of both genes enhances either effect, it can be assumed that, firstly, the P. anserina CLPP and i -AAA protease are involved in parallel pathways regulating lifespan and/or that their absence under standard growth conditions causes mild but tolerable stress leading to mitochondrial hormesis (that is, the beneficial activation of maintenance and repair pathways that ultimately results in the observed lifespan extension [21] ) and, secondly, that PaCLPP and PaIAP are cooperatively involved in a mitochondria-specific heat stress response. The underlying mechanisms, however, remain to be understood and have to be addressed in future studies. Similarly, the role of PaCLPX needs to be investigated in detail. As S. cerevisiae possesses a CLPX homologue despite the absence of CLPP [22] , it is probable that eukaryotic CLPX chaperones perform functions independent of their role in the CLPXP protease complex. Indeed, human CLPX has recently been shown to be involved in mitochondrial DNA maintenance through interaction with the mitochondrial transcription factor TFAM [23] . Comparative analysis of Δ PaClpP and a PaClpX deletion strain is likely to generate important insights into possible protease-independent functions of CLPX in P. anserina . Overall, the finding that deletion of PaClpP leads to an unexpected effect on lifespan, which can be reverted by human CLPP, identifies the potential of P. anserina to be used as an experimentally accessible system to study the yet unknown functions of eukaryotic CLP proteases, possibly including those of the human homologues. It thus may be possible to develop in vivo approaches for the characterization of substrate recognition mechanisms, to identify CLPXP-specific substrates, to unravel interactions of CLPXP with other components of the mitochondrial protein quality control system and to integrate the elaborated mechanisms into the complex molecular network of mitochondrial pathways governing development and biological ageing [1] , [2] , [3] . P. anserina strains and cultivation In the present study, the P. anserina wild-type strain ‘s’ [24] , the PaClpP deletion strain Δ PaClpP (ref. 10 ), the PaIap deletion strain Δ PaIap (ref. 17 ), a newly generated Δ PaClpP /Δ PaIap double deletion strain and a newly generated PaClpP deletion strain overexpressing human ClpP (Δ PaClpP / HsClpP _OEx) were used. All mutant strains are in the genetic background of the wild-type strain ‘s’. Strains were grown on standard cornmeal agar Biomalz-Mais-Medium (BMM) at 27 °C under constant light [25] . Lifespan determination To determine the lifespan of the strains used in this study, monokaryotic ascospores were isolated from independent crosses of the respective strains and germinated for 2 days at 27 °C in the dark on BMM supplemented with 60 mM ammonium acetate. After germination, pieces of the resulting 2 days old mycelia were placed on M2 agar race tubes (M2 medium: 0.25 g l −1 KH 2 PO 4 , 0.3 g l −1 K 2 HPO 4 , 0.25 g l −1 MgSO 4 × 7 H 2 O, 0.5 g l −1 urea, and 10 g l −1 yellow dextrin. Addition of 2.5 μg l −1 biotin, 50 μg l −1 thiamine, 5 mg l −1 citric acid × 1 H 2 O, 5 mg l −1 ZnSO 4 × 7 H 2 O, 1 mg l −1 Fe(NH 4 ) 2 (SO 4 ) 2 × 6 H 2 O, 2.5 mg l −1 CuSO 4 × 5 H 2 O, 25 μg l −1 MnSO 4 × 1 H 2 O, 50 μg l −1 Na 2 MoO 4 × 2 H 2 O, and 50 μg l −1 H 3 BO 4 after sterilization of the basal medium) and incubated at 27 °C under constant light. For lifespan determination under heat stress conditions, the isolates were allowed to grow for 2 days at 27 °C and then transferred to 37 °C (Heraeus BK 6160 climate chamber, Thermo Scientific) for the remainder of their life. The period of linear growth was recorded as lifespan in days. Growth rate was measured as growth of the mycelia in centimetres per day. Fertility analysis Assessment of female fertility was essentially performed as described previously [17] . Isolates of wild-type or Δ PaClpP , originating from monokaryotic ascospores, were grown on M2 agar plates at 27 °C under constant light for 13 days. To determine the ability of wild-type or Δ PaClpP to form fruiting bodies after exposure to heat stress, the same isolates were allowed to grow for eight days at 27 °C and then transferred to 37 °C (KBW 400 climate chamber, BINDER) for 5 days. Following spermatisation at day 13, all plates were incubated for an additional three days at 27 °C, after which the total number of perithecia developing on each plate was counted. The mean number of perithecia developing per plate overgrown with the wild-type strain ‘s’ at 27 °C or 37 °C was set as 100% female fertility. Measurement of growth rate under stress conditions To assess the susceptibility of Δ PaClpP to various oxidative stressors and dithiothreitol, monokaryotic ascospores were isolated from independent crosses of the wild-type and Δ PaClpP and germinated for 2 days at 27 °C in the dark on BMM supplemented with 60 mM ammonium acetate. After germination, pieces of the resulting 2 days old mycelia were placed on M2 agar plates supplemented with different concentrations of paraquat (0, 20, 80 or 150 μM), CuSO 4 (0, 100, 200 or 400 μM), H 2 O 2 (0, 0.04, 0.06 or 0.1%), or dithiothreitol (0, 0.5, 5 or 10 mM) and incubated at 27 °C under constant light. Plates containing H 2 O 2 were kept in the dark to protect hydrogen peroxide from degradation. Growth was recorded for 4 days and growth rate was measured as growth of the mycelia in centimetres per day. Cloning procedures and generation of P. anserina mutants The human ClpP cDNA open reading frame was amplified by PCR using the oligonucleotides BamHI-HsClpP_3 for (5′-TA GGATCC ATGTGGCCCGGAATATTG-3′) and XbaI-HsClpP_4rev (5′-AT TCTAGA TCAGGTGCTAGCTGGGAC-3′), introducing Bam HI and Xba I restriction sites (underlined). The amplicon was cloned into the pExMtterhph [10] backbone ( Bam HI/ Xba I digested) under control of the strong constitutive metallothionein promoter and the metallothionein terminator. The resulting plasmid pHsClpPEx1 was subsequently transformed into P. anserina Δ PaClpP spheroplasts. Transformants were selected for hygromycin B resistance and verified by Southern blot analysis. Strains containing a single integration of pHsClpPEx1 were termed Δ PaClpP / HsClpP _OEx. To construct a Δ PaClpP /Δ PaIap double deletion strain, a monokaryotic Δ PaClpP isolate was crossed with a monokaryotic Δ PaIap isolate. Meiotic offspring containing the concomitant deletion of both genes were identified by their phleomycin resistance and verified by Southern blot analysis. Production, regeneration and transformation of P. anserina spheroblasts The PaClpP deletion strain was grown on BMM at 27 °C under constant light for 3 days and subsequently under the same conditions in liquid complete medium for 2 days (complete medium: 3.7 g l −1 NH 4 Cl, 2 g l −1 tryptone, 2 g l −1 yeast extract, 10 g l −1 glucose, 1 g l −1 KH 2 PO 4 , 0.5 g l −1 KCl, 0.5 g l −1 MgSO 4 × 7 H 2 O, and 1 mg l −1 ZnSO 4 × 7 H 2 O, FeCl 2 × 4 H 2 O, and MnCl 2 × 2 H 2 O; pH 6.5). Twenty grams of the resulting mycelium were washed with TPS buffer (5 mM Na 2 HPO 4 , 45 mM KH 2 PO 4 , 0.8 M sucrose; pH 5.5) and TPS buffer containing 20 mg ml −1 Glucanex (Novozymes) was added to a final volume of 100 ml. After chopping the mixture in a Waring Blendor, the resulting suspension was incubated for 1.5 h at 35 °C. Following filtration through gauze and glass wool, the suspension was centrifuged for 10 min at 4,000 rpm to pelletize the spheroplasts and the pellet was washed three times with TPS buffer. To regenerate spheroplasts, the pellet was recovered in TPS buffer and the spheroplasts were plated on regeneration agar (3.7 g l −1 NH 4 Cl, 2 g l −1 tryptone, 1 g l −1 yeast extract 1 g l −1 casamino acids, 10 g l −1 glucose, 342.3 g l −1 sucrose, 1.5 g l −1 KH 2 PO 4 , 0.5 g l −1 KCl, 0.54 g l −1 MgSO 4 × 7 H 2 O, and 1 mg/l MnSO 4 × 1 H 2 O, FeSO 4 × 7 H 2 O, CuSO 4 × 5 H 2 O, and ZnSO 4 × 7 H 2 O; pH 6.0) containing 100 μg ml −1 hygromycin B. After 7–10 days of growth, mycelia of developing cultures were transferred to BMM agar plates. Integrative transformation of P. anserina spheroplasts was performed as described previously [26] . Southern blot analysis Total DNA of P. anserina was isolated following the protocol developed by Lecellier and Silar for rapid extraction of nucleic acids from filamentous fungi [27] . DNA digestion, gel electrophoresis and Southern blotting were performed according to standard protocols. For Southern blot hybridization and detection, Digoxigenin-labelled hybridization probes (DIG DNA Labelling and Detection Kit, Roche Applied Science) were used according to the manufacturer’s protocol. The HsClpP -specific hybridization probe was amplified by PCR using the oligonucleotides HsClpP_1for (5′-ATGTGGCCCGGAATATTG-3′) and HsClpP_2rev (5′-GCGAGTAGATGTCATAGG-3′) and corresponded to nucleotides 124-355 of the HsClpP cDNA (GenBank: BC002956.1). The PaClpP -specific hybridization probe corresponded to a 634-bp Pst I-fragment containing part of the PaClpP gene and its 3′-untranslated region. The PaIap -specific hybridization probe corresponded to a 1287-bp Nco I-fragment containing part of the PaIap gene. As a hybridization probe specific for the phleomycin resistance gene ( ble ), the 1293, bp Bam HI-fragment of the plasmid pKO3 ( [28] ) was used. Western blot and densitometry analysis Mitochondrial protein extracts from P. anserina strains were isolated according to a previously developed procedure [29] . Separation of proteins by SDS–PAGE and subsequent transfer of proteins to polyvinylidene difluoride (PVDF) membranes (Immobilon-FL, Millipore) were performed following standard protocols. Blocking and antibody incubation of blotted PVDF membranes were performed according to the Odyssey ‘Western Blot Analysis’ handbook (LI-COR). Primary antibodies were raised against a PaLON (UniProt: B2AZ54) synthetic peptide ([H]-CDKIGRGYQGDPS-[OH]; Sigma) corresponding to amino acids 677–688 (antibody dilution: 1:1,500), a PaCLPP (UniProt: B2B591) synthetic peptide ([Ac]-CGTMLSADAKEGKH-[OH]; NEP) corresponding to amino acids 242–254 (antibody dilution: 1:400) and the PaPORIN (UniProt: B2B736) full-length protein (NEP; antibody dilution: 1:5,000). The human CLPP antibody (abcam, product code: ab56455) was raised against an HsCLPP (UniProt: Q16740) recombinant fragment corresponding to amino acids 178–278 (antibody concentration: 1 μg ml −1 ). In all analyses, secondary antibodies conjugated with the infrared dyes IRDye 800CW or IRDye 680CW (LI-COR) were used (antibody dilution: 1:15,000). The Odyssey Infrared Imaging System (LI-COR) was used for detection and quantification was performed using the manufacturer's software as recommended. Blue native PAGE BN-PAGE was performed according to the protocol developed by Schägger and colleagues [18] . For sample preparation, 300 μg of mitochondrial protein extract was solubilised using a digitonin/protein ratio of 4:1 (w/w). Linear gradient gels (4–13%) overlaid with 3.5% stacking gels were used for separation of the solubilised samples. For western blotting of BN-PAGE gels, 0.05% SDS was added to the transfer buffer and the transfer was performed for 16 h at 25 V and 4 °C. Blocking, antibody incubation and antibody detection of blotted PVDF membranes were performed as described in the preceding section. Statistical analysis For statistical analysis of western blot data, two-tailed Student’s t -test was used. For statistical analyses of lifespan, growth rate and female fertility, two-tailed Wilcoxon rank-sum test was used. If not explicitly stated otherwise, the respective samples were compared with the appropriate wild-type sample. P -values<0.05 were considered statistically significant. How to cite this article: Fischer, F. et al . Human CLPP reverts the longevity phenotype of a fungal ClpP deletion strain. Nat. Commun. 4:1397 doi: 10.1038/ncomms2397 (2012).